Anomalous low-temperature Coulomb drag in graphene-GaAs heterostructures Vertical heterostructures combining different layered materials offer novel opportunities for applications and fundamental studies. Here we report a new class of heterostructures comprising a single-layer (or bilayer) graphene in close proximity to a quantum well created in GaAs and supporting a high-mobility two-dimensional electron gas. In our devices, graphene is naturally hole-doped, thereby allowing for the investigation of electron–hole interactions. We focus on the Coulomb drag transport measurements, which are sensitive to many-body effects, and find that the Coulomb drag resistivity significantly increases for temperatures <5–10 K. The low-temperature data follow a logarithmic law, therefore displaying a notable departure from the ordinary quadratic temperature dependence expected in a weakly correlated Fermi-liquid. This anomalous behaviour is consistent with the onset of strong interlayer correlations. Our heterostructures represent a new platform for the creation of coherent circuits and topologically protected quantum bits. Solid-state dipolar quantum liquids are many-particle systems of repulsively interacting dipoles made of electron–hole (e–h) pairs, which have been studied for the past 50 years (for recent reviews, see for example, refs 1 , 2 ). These systems display a rich and intriguing phenomenology. Particular attention has been devoted to the Bose–Einstein condensation (BEC) of e–h pairs, that is, exciton condensation, with notable results [1] , [2] . Optical signatures of BEC of excitons have been reported in optically excited exciton [3] , [4] , [5] and exciton–polariton [6] cold gases, where, however, non-equilibrium effects conflict, to some extent, with equilibrium thermodynamics. Spectacular implications of spontaneous coherence on transport have also been discovered in systems of permanent (interlayer) excitons [7] . Quantum Hall fluids in high-mobility GaAs/AlGaAs semiconductor double quantum wells display a large variety of transport anomalies [8] , [9] due to spontaneous coherence of interlayer excitons. There is an ongoing effort to find new systems that display spontaneous coherence and superfluidity of permanent excitons. In addition to the fundamental interest in understanding when these phenomena occur in nature, there is a practical interest in discovering many-particle systems where these types of orders occur under less extreme physical conditions, in particular in the absence of strong magnetic fields and, possibly, at non-cryogenic temperatures. Interest in interlayer excitons has been recently revitalized [10] , [11] , [12] by theoretical predictions of high-temperature spontaneous coherence and superfluidity in electrically decoupled graphene layers [13] , [14] , [15] and topological insulator thin films [16] , [17] , [18] , [19] . The former systems are just examples of van der Waals heterostructures [20] in which different layered materials are combined to offer novel opportunities for applications [21] , [22] , [23] and fundamental studies [10] , [11] , [12] . In the following, we report a new class of vertical heterostructures comprising a single-layer, SLG (or bilayer, BLG) graphene carrying a fluid of massless (massive) chiral holes in close proximity to a GaAs quantum well hosting a high-mobility two-dimensional (2D) electron gas. We focus on the Coulomb drag transport measurements, which are sensitive to many-body effects. We find that the Coulomb drag resistivity significantly increases for temperatures T <5–10 K, with a notable departure from the T 2 temperature dependence expected in a weakly correlated Fermi-liquid scenario [24] . The low-temperature data follow a logarithmic law, without the onset of saturation in the case of bilayer graphene/GaAs samples. This anomalous behaviour is consistent with the onset of strong interlayer correlations. These heterostructures may offer new routes for the exploration of a variety of e–h phenomena, including coherent circuits with minimal dissipation [25] , [26] , [27] and nanodevices including analogue-to-digital converters [28] and topologically protected quantum bits [29] . Sample design and characterization Our vertical heterostructures are prepared as follows: SLG and BLG flakes are produced by micromechanical exfoliation of graphite on Si/SiO 2 (ref. 30 ). The number of layers is identified by a combination of optical microscopy [31] and Raman spectroscopy [32] , [33] . The latter is also used to monitor the sample quality by measuring the D to G ratio [34] and the doping level [35] . Selected flakes are then placed onto a GaAs-based substrate at the centre of a pre-patterned Hall bar by using a polymer-based wet transfer process [22] (for details, see Supplementary Note 1 ). The GaAs-based substrates consist of modulation-doped GaAs/AlGaAs heterostructures hosting a 2D electron gas (2DEG) in the GaAs quantum well placed 31.5 nm below the surface. The heterostructures are grown by molecular beam epitaxy [36] and consist of a n -doped GaAs cap layer, a AlGaAs barrier, a GaAs well and a thick AlGaAs barrier with a delta doping layer (see Supplementary Fig. 1 ). Two different samples are fabricated: sample A, with a 15-nm-thick quantum well, and sample B, with a 22-nm quantum well. Hall bars (300 μm wide and 1,500 μm long) are fabricated by ultraviolet lithography. Ni/AuGe/Ni/Au layers are then evaporated and annealed at 400 °C to form Ohmic contacts to the 2DEG, to be used for transport and the Coulomb drag measurements (see Fig. 1 ). The Hall bar mesas are defined by conventional wet etching in acid solution. To ensure that the current in the 2DEG flows only in the region below the graphene flakes, channels with a width comparable to the transferred graphene flakes (typically ~30 μm) are defined in the Hall bar by electron beam lithography and wet etching ( Fig. 1e,f ). A SLG flake is transferred onto sample A and a BLG flake onto sample B. The integrity of the SLG and BLG flakes is monitored throughout the process by Raman spectroscopy. Supplementary Fig. 2 compares the Raman spectra of the as-prepared SLG on Si/SiO 2 and after transfer on GaAs. The analysis of G peak position, Pos(G), its full width at half maximum, FWHM(G), Pos(2D) and the area and intensity ratios of 2D and G peaks allow us to monitor the amount and type of doping [33] , [35] , [37] , [38] . This indicates a small p -doping for the as-prepared sample, decreasing to below 100 meV for the transferred sample [33] , [35] , [37] . The absence of a significant D peak both before and after transfer indicates that the samples have negligible amount of defects [33] , [34] and that the transfer procedure does not add defects. Similarly, no increase in defects is seen for the BLG samples. 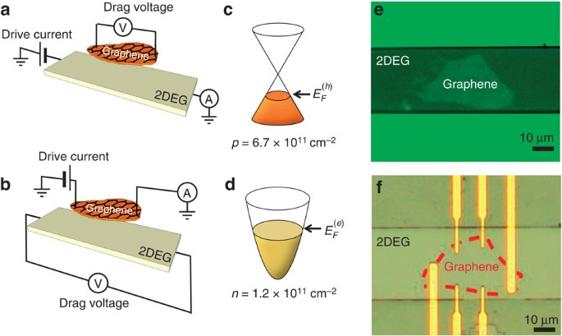Figure 1: Hybrid SLG/2DEG devices and the Coulomb drag transport set-up. (a,b) Configurations for the Coulomb drag measurements. Ina, a voltage dropVdragappears in graphene, in response to a drive currentIdriveflowing in the 2DEG. Inb, the opposite occurs. The drag voltage is measured with a low-noise voltage amplifier coupled to a voltmeter as a function of the applied bias. The drive current is also monitored. (c) Conical massless Dirac fermion band structure of low-energy carriers in SLG. The SLG in this work is hole-doped. (d) Parabolic band structure of ordinary Schrödinger electrons in the 2DEG. (e) Optical micrograph of the device before the deposition of Ohmic contacts. The SLG flake becomes visible in green light after the sample is coated with a polymer (PMMA)31. The scale bar is 10 μm long. (f) Optical microscopy image of the contacted SLG on the etched 2DEG GaAs channel. The red dashed line denotes the SLG boundaries. The scale bar is 10 μm long. Figure 1: Hybrid SLG/2DEG devices and the Coulomb drag transport set-up. ( a , b ) Configurations for the Coulomb drag measurements. In a , a voltage drop V drag appears in graphene, in response to a drive current I drive flowing in the 2DEG. In b , the opposite occurs. The drag voltage is measured with a low-noise voltage amplifier coupled to a voltmeter as a function of the applied bias. The drive current is also monitored. ( c ) Conical massless Dirac fermion band structure of low-energy carriers in SLG. The SLG in this work is hole-doped. ( d ) Parabolic band structure of ordinary Schrödinger electrons in the 2DEG. ( e ) Optical micrograph of the device before the deposition of Ohmic contacts. The SLG flake becomes visible in green light after the sample is coated with a polymer (PMMA) [31] . The scale bar is 10 μm long. ( f ) Optical microscopy image of the contacted SLG on the etched 2DEG GaAs channel. The red dashed line denotes the SLG boundaries. The scale bar is 10 μm long. Full size image To ensure that the 2D chiral hole gas in SLG/BLG and the 2DEG in GaAs are electrically isolated, we monitor the interlayer I I – V I characteristics in the T =0.25–50 K temperature range (see Supplementary Note 2 ), with I I and V I the interlayer (‘leakage’) current and interlayer voltage, respectively, and the layers being the SLG (or BLG) and the GaAs quantum well. In SLG-based devices, a negligible interlayer current <0.2 nA is measured for V I up to −0.3 V for all values of T , leading to interlayer resistances ~1 GΩ. In the case of BLG, for T ~45 K, I I increases to 100 nA at V I =−0.3 V, with the interlayer resistance increasing to several MΩ. In all cases, therefore, the interlayer resistance is much larger than the largest intralayer resistance for SLG, BLG and GaAs quantum well, which is ~10 kΩ. Magnetotransport and the Coulomb drag measurements To search for signatures of correlations between the 2DEG in the GaAs quantum well and the 2D chiral hole fluid [39] in SLG or BLG, we measure the T dependence of the Coulomb drag resistance R D . Experimentally, the Coulomb drag is routinely used as a sensitive probe of strong correlations including transitions to the superconducting state [40] , metal-insulator transitions [41] and Luttinger liquid correlations [42] in quantum wires, and exciton condensation in quantum Hall bilayers [9] . In a Coulomb drag experiment [24] , [43] , [44] , a current source is connected to one of the two layers (the active or drive layer). The other layer (the passive layer) is connected to an external voltmeter so that the layer can be assumed to be an open circuit (no current can flow in it). The drive current I drive drags carriers in the passive layer, which accumulate at the ends of the layer, building up an electric field. The voltage drop V drag related to this field is then measured. The quantity R D is defined as the ratio V drag / I drive and is determined by the rate at which momentum is transferred between quasiparticles in the two layers [24] . Before the Coulomb drag experiments, we performed magnetotransport measurements at 4 K, as for Fig. 2a,b . In our set-up, the 2DEG is induced in the quantum well by shining light from an infrared diode. In the SLG/2DEG device, we find a 2DEG with density n =1.2 × 10 11 cm −2 from low-field (below 1 T) classical Hall effect and a mobility μ e =13,000 cm 2 V −1 s −1 at 4 K. At T =45 K, the density decreases to 4.0 × 10 10 cm −2 and μ e =8,700 cm 2 V −1 s −1 . 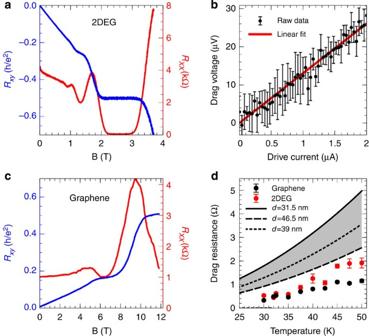Figure 2: Magnetotransport characterization of the 2DEG and SLG and high-temperature drag. (a,b) Hall resistanceRxy(blue solid line) and longitudinal resistanceRxx(red solid line) of 2DEG and SLG, respectively. Hall measurements are performed in the two layers with the same configuration of electrical connections: Hall resistance is positive for holes and negative for electrons. (c) Drag voltage in the 2DEG as a function of the drive current flowing in SLG atT=42.5 K: data and a linear fit are shown. Error bars are calculated as s.d. from the average of 10 current sweeps. (d) Drag resistanceRDas a function of temperature. Black (red) points refer toRDderived by measuring the voltage drop in SLG (2DEG), respectively. The three lines are Boltzmann-transport calculations in the Fermi-liquid regime (see ref.47andSupplementary Note 4). Different curves refer to different values of the interlayer distanced:d=31.5 nm (solid line), 46.5 nm (long-dashed line) and 39 nm (short-dashed line). Figure 2a ) shows the quantum Hall effect in the 2DEG. The quantum Hall plateaus at h /(2 e 2 ) and h /(4 e 2 ) (blue trace) correspond to the first two spin degenerate Landau levels [45] . In correspondence of the plateaus, minima are found [45] in the longitudinal resistance R xx (red trace). Figure 2: Magnetotransport characterization of the 2DEG and SLG and high-temperature drag. ( a , b ) Hall resistance R xy (blue solid line) and longitudinal resistance R xx (red solid line) of 2DEG and SLG, respectively. Hall measurements are performed in the two layers with the same configuration of electrical connections: Hall resistance is positive for holes and negative for electrons. ( c ) Drag voltage in the 2DEG as a function of the drive current flowing in SLG at T =42.5 K: data and a linear fit are shown. Error bars are calculated as s.d. from the average of 10 current sweeps. ( d ) Drag resistance R D as a function of temperature. Black (red) points refer to R D derived by measuring the voltage drop in SLG (2DEG), respectively. The three lines are Boltzmann-transport calculations in the Fermi-liquid regime (see ref. 47 and Supplementary Note 4 ). Different curves refer to different values of the interlayer distance d : d =31.5 nm (solid line), 46.5 nm (long-dashed line) and 39 nm (short-dashed line). Full size image The 2D chiral hole fluids in SLG and BLG have their highest mobility when the 2DEG is not induced. This is shown in Fig. 2b for the SLG-based device (see also Supplementary Note 3 ). Figure 2a,b indicates that the sign of the Hall resistance R xy in SLG is opposite to the 2DEG, thereby demonstrating that SLG is p -doped. At 4 K, the hole density is p =9.9 × 10 11 cm −2 and μ h =4,100 cm 2 V −1 s −1 . At 45 K, the corresponding values are p =6.7 × 10 11 cm −2 and μ h =2,400 cm 2 V −1 s −1 . Low- T magnetotransport in SLG ( Fig. 2b ) reveals quantum Hall plateaus at h /(2 e 2 ) and h /(6 e 2 ), corresponding to the massless Dirac fermions with spin and valley degeneracy [39] . On the contrary, when the 2DEG is optically induced, the hole density in SLG at 4 K is p =6.7 × 10 11 cm −2 and μ h =2,100 cm 2 V −1 s −1 , thereby weakening the manifestations of the quantum Hall effect (see Supplementary Fig. 3 ). The degradation of the SLG transport properties in the presence of the 2DEG could be linked to the creation of ionized Si donors within the n -doped GaAs cap layer, acting as positively charged scatterers [46] . We now focus on the Coulomb drag experiments. These are performed in the configuration sketched in Fig. 1a,b and in a 3 He cryostat with a 240 mK–50 K range. Ten V drag − I drive curves in a d.c. configuration are acquired for each T and then averaged. We first address the SLG/2DEG case. Figure 2c reports a representative set of averaged drag voltage data taken in the 2DEG at T =42.5 K. In this configuration, the SLG gating effect and consequent carrier depletion in the 2DEG are avoided by applying a positive current, from 0 to +2 μA in the SLG channel. Figure 2c ) shows that, at this representative T , the drag voltage is linear with the drive current, thereby allowing the extraction of R D from the slope of a linear fit. Figure 2d shows the plots of R D for 30 K≤ T ≤50 K, with the 2DEG used as the drive (black points) or passive (red points) layer. It also reports calculations of the temperature dependence of R D in a hybrid Dirac/Schrödinger SLG/2DEG double layer within a Boltzmann-transport theory, which is justified in the Fermi-liquid regime [47] , [48] . This is done by generalizing the theory of ref. 47 to include effects due to the finite width of the GaAs quantum well (see Supplementary Note 4 ). This shows that the experimental results in this temperature range are consistent with the canonical Fermi-liquid prediction [24] , [43] , [44] , [45] , [46] , [47] , [48] , [49] , [50] , that is, R D ∝ T 2 (see also Fig. 3a ), as constrained by the available phase-space of the initial and final states involved in the scattering process. The magnitude of the measured effect, however, is smaller than predicted by theory. Discrepancies of similar magnitude have been previously reported for the Coulomb drag measurements between two SLGs encapsulated in hexagonal boron nitride [11] . Figure 2d demonstrates that the Onsager reciprocity relations [51] , which in our case require that the resistance measured by interchanging drive and passive layers should not change, are satisfied in the 30 K≤ T ≤40 K range. A violation of reciprocity occurs for T >40 K. We ascribe this to the effect of the interlayer current I I , leading to an additional contribution sensitive to the exchange of active and passive layers (see Supplementary Note 2 and Supplementary Fig. 4 ). Consistent with this interpretation, we observe larger violations of Onsager reciprocity in the BLG/GaAs sample, where I I is three orders of magnitude larger than SLG/GaAs at T =45 K (see Supplementary Fig. 5 ). We now discuss the behaviour of R D in the low-temperature regime. We follow ref. 11 and use the lowest quality layer, in our case SLG, as the drive layer and measure the drag voltage in the 2DEG. In the reversed configuration, the drag voltage measured in SLG shows fluctuations [11] , [12] as a function of the drive current, which hamper the extraction of R D , see Supplementary Note 5 ). 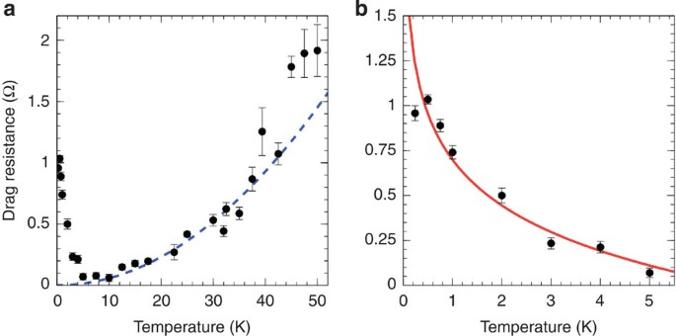Figure 3: Temperature dependence of the Coulomb drag resistance in the SLG/2DEG vertical heterostructure. (a)RDobtained from a linear fit of the measured voltage drop in the 2DEG (passive layer) as a function of the drive current flowing in the SLG (drive layer). Error bars are the s.d. as obtained in the fit procedure. The dashed blue line is a best-fit of the standard Fermi-liquid type24:RD(T)=aT2witha=(5.8±0.3) × 10−4ΩK−2. (b) Zoom ofRDin the low-Tlimit. The red solid line is a fit based on the functional form reported in equation (1). This fit describes very well theRDupturn at lowTas the system approachesTc~10–100 mK. (b) The data point at the lowest measuredT=240 mK deviates from the logarithmic trend, possibly pointing to the onset of a saturation effect. R D measured in the 2DEG reveals an anomalous behaviour below 10 K. Figure 3 indicates that R D deviates from the ordinary T 2 dependence, as shown by a large upturn for T lower than an ‘upturn’ temperature T u ~5 K. The enhancement of R D at low T is a very strong effect: the drag signal increases by more than one order of magnitude by decreasing T below T u , where R D is vanishingly small, in agreement with the Fermi-liquid predictions (see Supplementary Note 4 ), down to T =240 mK. Figure 3: Temperature dependence of the Coulomb drag resistance in the SLG/2DEG vertical heterostructure. ( a ) R D obtained from a linear fit of the measured voltage drop in the 2DEG (passive layer) as a function of the drive current flowing in the SLG (drive layer). Error bars are the s.d. as obtained in the fit procedure. The dashed blue line is a best-fit of the standard Fermi-liquid type [24] : R D ( T )= aT 2 with a =(5.8±0.3) × 10 −4 ΩK −2 . ( b ) Zoom of R D in the low- T limit. The red solid line is a fit based on the functional form reported in equation (1). This fit describes very well the R D upturn at low T as the system approaches T c ~10–100 mK. ( b ) The data point at the lowest measured T =240 mK deviates from the logarithmic trend, possibly pointing to the onset of a saturation effect. Full size image Figure 3b is a zoom of the drag enhancement data in the low- T range together with a fit (solid line) of the type: where R 0 and A are two fitting parameters and T c indicates the mean-field critical temperature of a low- T phase transition at which the drag resistance would display a weak singularity. This fitting procedure cannot predict T c : for example, fixing T c =10 mK, the best-fit yields A =(0.416±0.015) Ω and R 0 =(2.66±0.08) Ω. We can well fit the experimental data by choosing any value of T c , as long as this is substantially lower than the lowest investigated temperature, that is, T =240 mK. As it is clear from the functional form of the fitting function in equation (1), in this regime a change can be reabsorbed into a change of the background resistance . Despite this caveat, we note that our fitting procedure is in excellent agreement with the data for T c in the range 10–100 mK. We note, however, that the data point at the lowest measured T =240 mK deviates from the logarithmic trend, possibly pointing to the onset of saturation. To further investigate this, we explore a second device comprising of a hole-doped exfoliated BLG deposited on the surface of a GaAs quantum heterostructure. The hole density in BLG is p =1.4 × 10 12 cm −2 from the low-field (below 1 T) classical Hall effect and the mobility is 670 cm 2 V −1 s −1 at 4 K. The 2DEG has an electron density n =2 × 10 11 cm −2 and a mobility 86,000 cm 2 V −1 s −1 at 4 K. Contrary to the SLG/2DEG case, in the BLG/2DEG device, both electron and hole fluids have parabolic energy–momentum dispersions ( Fig. 4b,c ). A lower kinetic energy in BLG (vanishing like k 2 (ref. 39 ) rather than like k for small values of momentum ℏ k ) compared with SLG is expected to enhance the relative importance of Coulomb interactions [52] . It is therefore interesting to evaluate whether this enhancement manifests in the low-temperature drag resistance. To probe this, we measure the evolution of R D as a function of T using BLG as the drive layer ( See Supplementary Figs. 6 and 7 ). 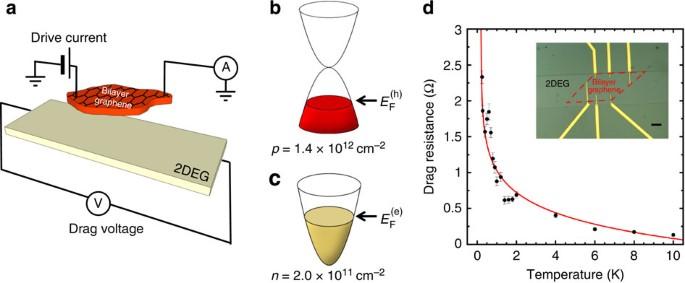Figure 4: Temperature dependence ofRDin the BLG/2DEG vertical heterostructure. (a) Configuration for the Coulomb drag measurements. A voltage dropVdragappears in the 2DEG in response to a currentIdrivethat flows in BLG. (b) Low-energy parabolic band structure of massive chiral holes in BLG39. (c) Parabolic band structure of Schrödinger electrons in the 2DEG. (d)RDin the low-Tlimit. The red solid line is a fit based on the functional form reported in equation (1) withTc~190 mK. Contrary to the SLG/2DEG case, no signal of saturation is observed down to the lowest values ofT. The inset shows an optical microscopy image of the contacted BLG on the etched 2DEG GaAs channel. The red dashed line denotes the BLG boundaries. The scale bar is 10 μm long. Figure 4 again shows a significant departure from the Fermi-liquid T 2 dependence. Consistent with the expected larger impact of interactions [52] , [53] , we get T u ~10 K, that is, twice the SLG/2DEG case, while the best-fit of R D data based on equation (1) yields T c =190 mK (to be compared with T c =10–100 mK in the SLG/2DEG). The observed drag resistance remains two–three orders of magnitude smaller than the layer resistance. However, if we follow the logarithmic increase of the drag signal as T approaches T c , the drag resistance can reach arbitrarily large values, of the order of 10 2 –10 3 Ω (that is, comparable to the isolated-layer resistance). Figure 4: Temperature dependence of R D in the BLG/2DEG vertical heterostructure. ( a ) Configuration for the Coulomb drag measurements. A voltage drop V drag appears in the 2DEG in response to a current I drive that flows in BLG. ( b ) Low-energy parabolic band structure of massive chiral holes in BLG [39] . ( c ) Parabolic band structure of Schrödinger electrons in the 2DEG. ( d ) R D in the low- T limit. The red solid line is a fit based on the functional form reported in equation (1) with T c ~190 mK. Contrary to the SLG/2DEG case, no signal of saturation is observed down to the lowest values of T . The inset shows an optical microscopy image of the contacted BLG on the etched 2DEG GaAs channel. The red dashed line denotes the BLG boundaries. The scale bar is 10 μm long. Full size image The observed upturn of the drag resistance as a function of T is puzzling and so is the fact that the experimental data in the upturn regime are well fitted by a logarithmic function, rather than an exponential or a power law. We now elaborate on possible explanations of this phenomenology. Ref. 54 [54] predicted a finite value of the drag resistivity at T =0 as a consequence of higher-order effects in perturbation theory (third order in the interlayer interaction). The predicted value of interaction-induced drag, however, is far too small (≈10 −5 Ω per square) to explain our upturn. Mesoscopic effects can lead both to positive and negative fluctuations of the low-temperature drag resistivity as a function of the electron density [55] . In our experiments, however, the upturn is fully reproducible for different devices (SLG/GaAs and BLG/GaAs) and cool downs (yielding slightly different densities). We therefore exclude that this effect is responsible for the logarithmic increase. Finally, the disorder effects in the diffusive regime [49] , [50] do lead to a logarithmic enhancement of the drag signal of the form R D ( T ) ∝ − T 2 log( T ) for T →0, which is therefore a correction to the Fermi-liquid behaviour and not an upturn. The logarithmic enhancement of R D described by equation (1) was theoretically predicted in refs 17 , 18 on the basis of a Boltzmann-transport theory for e–h double layers, where the scattering amplitude is evaluated in a ladder approximation [56] . Similar results were obtained on the basis of a Kubo-formula approach [57] . Within these frameworks, the enhancement is attributed to e–h pairing fluctuations extending above T c for a phase transition into an exciton condensed phase [1] , [17] , [18] , [57] , [58] . If this scenario is correct, Fig. 3b indicates that the T range above T c , in which fluctuations are responsible for deviations from the Fermi-liquid T 2 dependence, is very large. This can be ascribed to the quasi-2D nature of our SLG/2DEG heterostructure and shares similarities with other 2D systems where fluctuations play an important role, such as cuprate superconductors (see, for example, ref. 59 ) and ultracold Fermi gases [60] . The mismatch in the Fermi wave numbers , which is ~25% in the SLG/2DEG and Δ k F ~30% in the BLG/2DEG case, raises concern on the validity of the exciton-condensate scenario. (Here and are the Fermi wave numbers in the layers with n - and p -doping, respectively.) Indeed, such a mismatch is expected [61] to weaken the robustness of the exciton-condensate phase in which the condensed e–h pairs have zero total momentum ℏ K . However, preliminary calculations including screening in the condensed phase [62] , [63] , [64] indicate that the K =0 exciton-condensate state persists even in the presence of these values of Δ k F , with T c scales comparable to those reported here. On the other hand, a mismatch in the Fermi wave numbers of the two fluids may favour Fulde–Ferrell–Larkin–Ovchinnikov [65] or Sarma [66] phases. These are however rather fragile in dimensionality d >1, although evidence of a Fulde–Ferrell–Larkin–Ovchinnikov phase was reported, for example, in the layered heavy-fermion superconductor CeCoIn 5 (ref. 67 ). We stress that a perfect matching condition would be essential for the exciton-condensate scenario if the system was in the BCS weak-coupling regime, where a small density imbalance leads to a chemical potential difference greater than the pairing gap, and this would indeed destroy superfluidity. However, it was shown theoretically that e–h superfluidity can only appear at experimentally reachable temperatures when the system is already in the so-called BCS–BEC crossover [64] . In this regime, superfluidity is robust against density imbalance, and there is strong evidence from both theory and experiment [61] , [68] , [69] that it is not killed by the Fermi surface mismatches up to 50%. Finally, we recall that upturns of the Coulomb drag resistivity were reported in e–h doped GaAs/AlGaAs coupled quantum wells [70] , [71] , [72] . However, the combination of 2D electron and hole gases in the same GaAs material required a large nanofabrication effort, and the reported magnitude of the drag anomalies was smaller than in our hybrid heterostructures. Our observations establish a new class of vertical heterostructure devices with a potentially large flexibility in the design of band dispersions, doping and e–h coupling, where excitonic phenomena are accessible. How to cite this article : Gamucci, A. et al . Anomalous low-temperature Coulomb drag in graphene-GaAs heterostructures. Nat. Commun. 5:5824 doi: 10.1038/ncomms6824 (2014).